Growth rates of Florida corals from 1937 to 1996 and their response to climate change Ocean acidification causes declines in calcification rates of corals because of decreasing aragonite saturation states (Ω arag ). Recent evidence also indicates that increasing sea surface temperatures may have already reduced growth and calcification rates because of the stenothermic threshold of localized coral populations. Density banding in coral skeletons provides a record of growth over the coral's lifespan. Here we present coral extension, bulk density and calcification master chronologies from seven subtropical corals ( Montastraea faveolata ) located in the Florida Keys, USA with a 60-year common period, 1937–1996. Linear trends indicate that extension increased, density decreased and calcification remained stable while the most recent decade was not significantly different than decadal averages over the preceding 50 years for extension and calcification. The results suggest that growth rates in this species of subtropical coral have been tolerant to recent climatic changes up to the time of collection (1996). Ocean acidification due to rising atmospheric carbon dioxide ( p CO 2,air ) is cited as a threat to calcifying marine organisms [1] , [2] , [3] , [4] , [5] , [6] , [7] , [8] , [9] , [10] . When ocean acidification is combined with physiological stress from rising sea surface temperatures (SSTs), shifts in community structure and accelerating degradation of coral reef ecosystems may result [11] , [12] , [13] , [14] . The impacts of ocean acidification and SST on calcification rates remain topics of some debate [15] , [16] , [17] , [18] , [19] , [20] . The projected trend of future ocean acidification and SST rise [21] , [22] is expected to increasingly inhibit the calcifying potential of marine organisms in the near future [1] , [2] , [3] , [4] , [5] , [6] . However, taxa-specific calcification response [23] , [24] and the spatial and temporal variability in ocean acidification [6] , [25] , [26] , [27] are likely to regionally modify predicted declines in calcification rates. Historical declines in calcification are estimated at ∼ 10% for the twentieth century with declines in calcification predicted to double during the twenty-first century [10] , [28] . Many experimental studies demonstrate that reductions in pH and carbonate ion (CO 3 2− ) concentration (similar to that expected because of increasing p CO 2,air ) cause substantial and predictable declines in coral calcification [29] , [30] . These laboratory results are based on constraining limiting factors to known values of pH, aragonite saturation states (Ω arag ) or concentration of CO 3 2− . In situ coral calcification is subject to complex interactions of limiting environmental variables such as temperature, light, nutrients and water chemistry; however, comparably few laboratory studies account for these interactions [31] , [32] , [33] , [34] . Cyclic variations in skeletal porosity of many corals produce annual density bands [35] that provide a record of linear extension, bulk density and calcification. Identifying limiting environmental variables of coral growth is an aim of effective coral sclerochronology; however, individual variables commonly explain only a portion of the annual variability in growth rates. Multidecadal growth records from the Pacific spanning the twentieth century initially demonstrated a positive linear relationship between annual calcification and SST across a latitudinal range [36] and over time (through 1990), with SST accounting for roughly 30% of the annual variability and indicating a ∼ 4% increase in calcification per 1 °C [37] , [38] , [39] . More recently, declines in extension and calcification over the past two decades (ca 1985–2005) from the Pacific, Andaman Sea and Red Sea have primarily been attributed to increased SST suggesting the relationship is nonlinear, where both low and high temperatures are capable of reducing growth rates [39] , [40] , [41] , [42] , [43] . In contrast, a linear negative relationship between extension rate and SST was reported for a 440 years coral record from the Bahamas and accounted for 45% of the variability in extension rates based on 6-year timescales [44] . Declines in annual density and calcification were reported from 1934 to 1982 based on 35 Porites corals from the Great Barrier Reef (GBR) [38] ; however, more recent temporal models, constructed from 328 GBR corals, indicated that extension and calcification increased from 1900 to 1970 and first began to decline from 1990 to 2005 [41] . No significant trend was present in extension or calcification from 1801 to 1990 for a single Porites coral from French Polynesia [37] . Declines in extension (30%) and calcification (18%) were reported in Red Sea corals ( Diploria heliopora ) from 1998 to 2008 relative to the 1976–1997 mean values [43] . Examination of long-term coral growth records from the literature suggest that growth trends have not consistently exhibited the long-term linear declines in calcification expected from ocean acidification over the extent of twentieth century and that the measured declines in growth have been limited to recent decades and largely attributable to increasing SST. In this paper, we report on the trends, variability and decadal averages of historical coral growth records in relation to climate change and ocean acidification. The growth data are analysed against environmental variables, climatic/oceanic indices and modelled estimates of Ω arag . The historical changes and projected trends in SST and Ω arag are thought to have already limited coral growth or soon to be limiting controls on coral growth rates. Although declining coral growth is becoming more apparent world-wide, these growth data from subtropical reefs of the Florida Keys indicate a unique historical response of sustained calcification rates and increasing extension rates up to 1996. Growth rates of Florida corals Annual extension, density and calcification data are presented from seven coral cores of Montastraea faveolata colonies collected in the upper Florida Keys, USA, in May 1997 and June 1998. Over the 60-year period, 1937–1996, mean annual linear extension is 0.79±0.07 cm per year, mean annual bulk density is 1.18±0.06 g cm −3 and mean annual calcification is 0.91±0.06 g cm −2 per year. The coefficient of variation (CV) demonstrates the variability of annual values over time (inter-annual variability) irrespective of differences in the means. The CV in extension was 20% (range of individual cores: 15–24%), density was 11% (7–16%) and calcification was 17% (14–23%). The CV of growth parameters are similar to those for Porites from the GBR, in which density (6–9%) is the most conservative and extension (28–31%) and calcification (28–30%) are more variable [38] , [40] . The combination of extension, density and calcification measurements provides the most complete perspective of coral growth variability [45] . The relationship between the growth parameters over the 60-year record indicates that extension was negatively related to density ( r= −0.72, P <0.01, n =60), extension was positively related to calcification ( r= 0.72, P <0.01, n =60) and no significant relationship was present between calcification and density ( r= −0.07, P =0.62, n =60), which is in agreement with other coral growth studies [36] , [38] , [45] , [46] . Trends based on the linear regressions of the standardized anomaly data (STDA; Fig. 1 ) indicated a significant increase in extension rates ( P =0.048, n =60), a significant decrease in skeletal density ( P <0.001, n =60) and no significant change in calcification rates ( P =0.395, n =60). Coefficients of determination ( r 2 ) for linear regression of the growth data are low because of the high inter-annual variability of growth parameters and indicated that a linear regression poorly explained the annual variability in growth parameters. For this reason, it is useful to assess the growth data as decadal averages ( Fig. 2 ). No significant differences were present between the decadal averages beginning with 1937–1946 and ending with 1987–1996 for extension or calcification rates (single-factor analysis of variance at P <0.05, n =10). Significant differences were present in decadal averages of density data; most notably, the decade 1977–1986 was significantly lower than the other five decades ( t -test at P <0.01, n =10), whereas density of the most recent decade 1987–1996 was not significantly lower than the preceding five decades. 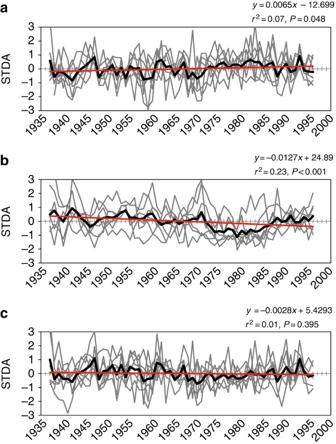Figure 1: Coral growth master chronologies 1937–1996. Master chronologies (n=7 corals) are presented in standardized anomaly (STDA) units for the period of 1937–1996 and depicted by bold black lines with the individual coral records comprising the master chronology depicted by grey lines. Linear regression lines for the master chronology data are depicted by red lines. Annual linear extension (a) exhibits a slight, but significant increasing trend. Annual skeletal bulk density (b) exhibits a significant decreasing trend. Annual calcification (c) exhibits no significant trend over the 60-year period. Figure 1: Coral growth master chronologies 1937–1996. Master chronologies ( n =7 corals) are presented in standardized anomaly (STDA) units for the period of 1937–1996 and depicted by bold black lines with the individual coral records comprising the master chronology depicted by grey lines. Linear regression lines for the master chronology data are depicted by red lines. Annual linear extension ( a ) exhibits a slight, but significant increasing trend. Annual skeletal bulk density ( b ) exhibits a significant decreasing trend. Annual calcification ( c ) exhibits no significant trend over the 60-year period. 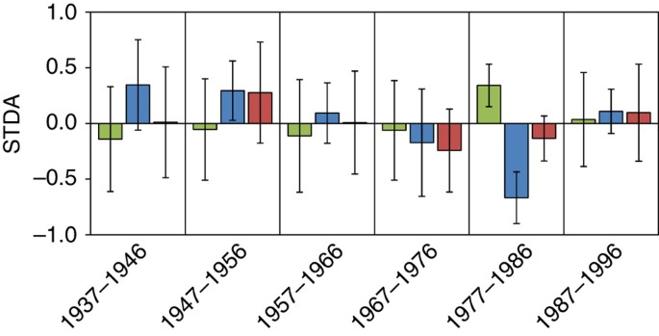Figure 2: Decadal coral growth averages. Decadal averages from master chronologies of annual extension in green, density in blue and calcification in red are presented in standardized anomaly (STDA) units with error bars representing the standard deviation for each decade (n=10). Full size image Figure 2: Decadal coral growth averages. Decadal averages from master chronologies of annual extension in green, density in blue and calcification in red are presented in standardized anomaly (STDA) units with error bars representing the standard deviation for each decade ( n =10). Full size image Coral growth and environmental correlates Coral growth master chronologies are compared with environmental and climatic records consisting of SST, rainfall, modelled Ω arag , Atlantic multidecadal oscillation (AMO) [47] and North Atlantic oscillation (NAO) [48] indices. Correlation of growth parameters with SST indicated significant positive relationships between calcification and annual average temperature and minimum monthly temperature, but no significant relationship to maximum monthly temperature ( Table 1 ). Annual SST for the study site exhibited no significant linear trend over the period 1937–1996 ( r 2 =0.05 P =0.087, n =60). 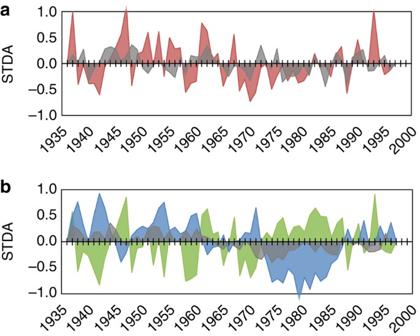Figure 3: Coral growth and environmental correlates. Coral growth parameters are plotted against environmental correlates. Ina, annual calcification is depicted in red as standardized anomaly (STDA) units and is positively related to the annual sea surface temperature anomaly depicted in grey. Inb, annual density, depicted in blue, is positively related to the AMO index, depicted in grey, whereas annual extension, depicted in green, is negatively related to the AMO index. Figure 3 illustrates the intermittent agreement between annual calcification anomaly and annual temperature anomaly. Rainfall was not significantly related to extension, density and calcification, nor was the NAO significantly correlated to any of the growth parameters on annual scales. Table 1 Correlation of growth parameters with environmental records. Full size table Figure 3: Coral growth and environmental correlates. Coral growth parameters are plotted against environmental correlates. In a , annual calcification is depicted in red as standardized anomaly (STDA) units and is positively related to the annual sea surface temperature anomaly depicted in grey. In b , annual density, depicted in blue, is positively related to the AMO index, depicted in grey, whereas annual extension, depicted in green, is negatively related to the AMO index. 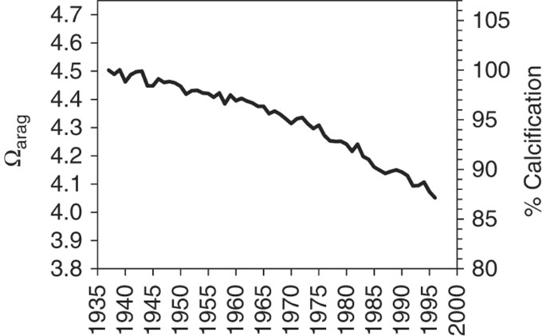Figure 4: Aragonite saturation state and calcification. Modelled aragonite saturation state, Ωarag, (leftyaxis) is presented for the period of the coral growth record (1937–1996) encompassing the study site (24°–25° N and 80°–81° W) along with the calculated percent change in calcification (rightyaxis) assuming 100% calcification in 1937. Full size image Modelled values of aragonite saturation state are presented in Figure 4 along with the predicted response in calcification based on an assumption of 100% calcification in 1937, which declines by 13% through 1996. The measured calcification data ( Fig. 1 ) failed to demonstrate this decline and was not significantly correlated with Ω arag on an annual basis ( r =0.09, P= 0.517, n= 60). Extension was negatively related to Ω arag , though non-significantly ( r =−0.25, P= 0.057, n= 60). Density was the only growth parameter that exhibits a significant correlation with Ω arag ( r =0.42, P <0.001, n =60). Figure 4: Aragonite saturation state and calcification. Modelled aragonite saturation state, Ω arag , (left y axis) is presented for the period of the coral growth record (1937–1996) encompassing the study site (24°–25° N and 80°–81° W) along with the calculated percent change in calcification (right y axis) assuming 100% calcification in 1937. Full size image The AMO exhibited a significant positive relationship with density ( r =0.57, P <0.001, n =60) explaining 33% of the annual variability. The AMO was negatively related to extension ( r =−0.25, P =0.050, n =60) and positively related to calcification ( r =0.19, P =0.151, n =60). The relationship between extension, density and the AMO is presented in Figure 3 and illustrates the positive relationship between the density anomaly values (negative relationship for extension) and the positive phase (1937–1965) and negative phase (1965–1996) of the AMO. The growth records from these subtropical corals do not exhibit significant declines in calcification or extension on the basis of linear trends or decadal averages. Age effects on coral growth [39] , on the basis of 43 Porites records over at least 100 years, indicate that extension may increase by time and density and may decrease by time independent of environmental trends such as increasing SST or decreasing Ω arag ; whereas, calcification exhibits no detectable age effect through time. In this study, annual extension exhibited a significant increase and annual density exhibited a significant decrease over the 60-year period based on linear trends. However, following methods for determining age effects [39] , the 10-year averages of the seven cores in this study with start years between 1906 and 1937, show no evidence of significant age effects over a 60-year period for extension ( y =0.0072 x +0.7635, r 2 =0.388, P =0.186), density ( y =−0.0041 x +1.211, r 2 =0.0822, P =0.582) or calcification ( y =0.0023 x +0.9133, r 2 =0.0282, P =0.750). Considering the annual variability in extension and calcification of these coral records, change over time is best assessed by evaluating the combination of long-term variability, trends and decadal averages, rather than the difference between the mean values of individual years. For example, the difference in annual calcification between the years 1937 and 1996 represents a 15% decline in calcification; however, this change is neither supported by a significant linear trend nor by significant differences between decadal averages. The lack of declines in extension or calcification does not necessarily suggest that corals or coral reefs at this study site are healthy [49] , but rather demonstrates that the measured corals have historically been able to maintain rates of extension and calcification over the 60-year period from 1937 to 1996 under the combination of local environmental and climatic changes. The subtropical location of these reefs may contribute to their persistent ability to grow and calcify under less than optimal environmental conditions. The lack of decline in coral extension and calcification rates raises important questions as to whether these corals exhibit a particularly high tolerance to changing conditions, whether the subtropical location of these corals is not representative of global estimates of past environmental or climatic change and variability, or whether environmental variables have yet to cross critical thresholds for sustaining coral growth and calcification. Calcification rates were positively related to SST, similar to results of Porites corals from Tahiti [37] and the GBR [38] ; however, SST only explained about 7% of the annual variability in calcification of these corals as opposed to ∼ 30% for the Pacific locations. A negative response to high SST [39] , [40] , [41] , [42] , [43] was not present up to 1996, although this does not preclude a potential negative response associated with the 1997–1998 mass-bleaching event that affected corals in this region [50] . Although the ability of these subtropical corals to calcify and grow has not been limited as of 1996, it is important to note that extreme events such as bleaching or disease outbreaks have led to widespread mortality in spite of otherwise sustainable growth conditions. The lack of a significant positive relationship between Ω arag and extension or calcification, or significant declines in extension and calcification, suggest that estimated declines in Ω arag have not, as of 1996, measurably limited the ability of these subtropical corals to accrete skeletal material (calcification) or construct new skeletal structures (extension). The decline in skeletal density over this period may suggest changes in how the corals are constructing the skeleton. The inter-annual variability of Ω arag (CV=3%) does not appear to be a dominant limiting environmental factor controlling the large annual variations in growth parameters (CV=11–17%). It is useful to consider that the modelled Ω arag data are based on oceanic parameters, which could differ substantially within the coastal zone and may not accurately describe the near-reef carbonate chemistry dynamics; nevertheless, the lack of declines in extension and calcification suggests that the global oceanic secular declines of Ω arag are not reflected in the calcification and growth of these subtropical corals over time. The positive relationship between density and Ω arag could suggest a weakening of coral skeleton in response to declines in Ω arag over time; however, a corresponding reduction in calcification is not present. Skeletal density is the quotient of variations in the amount of skeletal accretion (calcification) and the rate of upward growth (extension). Considering the opposite linear trends in density and extension and the lack of significant trend in calcification, it seems that the decline in density is the result of increasing extension over time, as opposed to potential declines in the calcification of these corals. A stretching modulation response [51] , in which corals exposed to higher environmental stress respond by increasing extension although maintaining calcification with a resulting decrease in skeletal density, may provide an alternative interpretation to the increased extension. However, the concept of stretching modulation was based on the response of corals, from different locations, to increasing stress along a spatial gradient, whereas the corals in this study exhibit changes in extension and density on a temporal basis. It could be inferred that increasing extension and decreasing density indicate a response to potentially increasing environmental stress (that is, declining Ω arag ) over time. If this stress response was responsible for the linear trends over time, it would be expected that the most recent decade (1987–1996) would have the highest extension rate and the lowest density; however, as illustrated in Figure 2 , this is not the case. Influence of the AMO on surface climate and weather varies regionally, but a positive phase is generally characterized by warmer temperatures and increased rainfall over Florida along with increased Atlantic hurricane activity [47] , [52] . The high correlation between density and the AMO might suggest that large-scale oceanic and climatic cycles are driving the variability in extension and calcification based on complex interactions of temperature, rainfall and related affects from cloud cover, storm activity and light availability that can vary on seasonal, annual and decadal timescales, and which are ultimately reflected in the skeletal density. Because of the multidecadal cycle of the AMO, it is not possible to test the agreement of multiple phases using a 60-year coral record; however, considering that the AMO shifted back to a positive phase in the mid 1990s, it may be posited that growth parameters would return to levels similar to those from 1937 to 1957 (that is, higher skeletal density, lower extension rates and neutral to higher calcification rates) and on the basis of the decadal growth averages this seems to be a reasonable hypothesis. Previous coral growth studies [53] , [54] in the upper Florida Keys consisted only of extension rates and generally agree with the relationship to AMO cycles presented in this paper. Extension rate data from Biscayne National Park [54] were at or below average from 1860 to 1880 (positive AMO), above average from 1880 to 1940 (negative AMO), below average and declining from 1940 to 1965 (positive AMO) and below average, but increasing from ∼ 1965 to the end of the record in 1984 (negative AMO). Extension data from Key Largo were reported as 5-year averages [53] and exhibited a general decreasing trend from 1953 to 1968 (positive AMO) and a general increasing trend from 1968 to 1978 (negative AMO). However, without accompanying calcification and density data, which exhibits the highest correlation to the AMO in the present study, it is difficult to draw strong conclusions about AMO and coral growth relationships. Considering the potential threats from rising temperatures and ocean acidification, there are two fundamental explanations for the increasing extension and stable calcification over the 1937–1996 period at this location: the degree of change in SST, rainfall, Ω arag and AMO at this study site was insufficient to limit the growth potential of these corals or the measured corals were capable of tolerating these changes in environmental and climatic variables. The AMO represented the strongest environmental correlate with coral growth parameters and it would be useful to assess this relationship over multi-century coral records, which pre-date recent global warming and rise in carbon dioxide to determine the potential long-term natural variability associated with the AMO. Relative to ocean acidification, these Florida Keys corals maintained their rates of calcification through 1996, despite the expected declines in calcification based on modelled Ω arag . Explanations for the lack of decline in calcification over time as expected from ocean acidification could be that: massive reef-building corals are not as susceptible to declines in Ω arag (ref. 55 ) as demonstrated by laboratory experiments; local process, such as high seasonal variation in Ω arag in the Florida Keys [25] , may be temporarily enabling these corals to maintain their historical rates of calcification; the role of Ω arag in controlling calcification is masked amidst considerable natural inter-annual variability; or the actual in situ reef-site carbonate chemistry is decoupled from the oceanic values, which could occur as a result of shifts in benthic community metabolism, mineral buffering and/or coastal biogeochemical processes. Ongoing retrospective monitoring of coral growth rates from existing cores and updated coral core records is necessary to better identify growth rate changes over time associated with potential local variability across the Florida reef tract and ultimately to identify large-scale variability throughout the western Atlantic, Caribbean and Gulf of Mexico. Coral samples and X-radiography Coral cores collected in May 1997 and June 1998 from seven Montastraea faveolata colonies located in the upper Florida Keys, USA, (24°–25° N and 80°–81° W) were drilled at the location of maximum vertical growth of the colony using a hydraulic drill with 10-cm-diameter barrel. Cores were sectioned into 0.4–0.7 cm-thick parallel-sided slabs oriented along the primary growth axis, based on the orientation of corallites on the sample surface. Slabs were X-rayed on Kodak Industrex AA400 8×10 Ready-pack II film (Kodak) using a self-rectified dental X-ray machine with settings of 70 kV and 15 mA, a source to object distance of 1.5 m and exposure times of 5–10 s. Films were manually developed and digitized with a medical film scanner at the native resolution of the CCD, which was 357 d.p.i. Digitized X-radiographs were assembled into a mosaic image for the entire core. Chronologies were constructed from the annual density bands and it was determined that all cores had a 60-year common period from 1937 to 1996. Coral densitometry and growth measurements Coral growth parameters were measured from digitized X-radiographs based on a process of relative optical densitometry [45] , [56] using a computer programme, CoralXDS+ ( http://www.nova.edu/ocean/coralxds/index.html ). Relative optical densitometry is based on the premise that when two materials (for example, a coral sample and an aluminium standard) are X-rayed and the exposed film exhibits equal optical density for both materials, the density of the sample material can be calculated [56] , [57] from: where τ ms is the relative mass absorption coefficient of the sample, τ mst is the relative mass absorption coefficient of the standard, ρ s is the density of the sample, ρ st is the density of the standard, η s is the thickness of the sample and η st is the thickness of the standard. Solving for the density of the coral sample yields For a given working range of exposure parameters, τ mst / τ ms can be converted to a constant relative mass absorption coefficient ratio and the value τ mr substituted: Hence, the density of the coral sample (skeletal bulk density) can be determined if the relative mass absorption coefficient ratio, density of the standard and thicknesses of the sample and standard are known. The τ mr was determined to be 0.622 by plotting relative optic density curves along the lengths of an aluminium wedge ( Al ) and a Tridacna aragonite wedge ( Ar ) against ρη and determining the τ mr value that produced the lowest residual difference, calculated as Σ|( τ mr Al − Ar )|. The aluminium wedge standard (density=2.7029 g cm −3 , length=5.1629 cm, height=0.9975 cm and slope=−0.1743) was included in all X-radiographs and used for density calibration. Using the CoralXDS+ program, a transect running normal to the orientation of density bands was selected on the coral X-radiograph image. The pixels within the transect were converted to skeletal bulk density, averaged over the width of the transect and plotted as a function of distance along the length of the transect. High-density, low-density and annual bands were determined by the second derivative zero crossing (inflection point) of a cubic spline of the density transect data. Bulk density was measured in g cm −3 , linear extension was measured in cm per year and calcification, in g cm −2 per year, was calculated from the product of extension and density. Master chronologies of extension, density and calcification were constructed from STDA in which the mean growth over the common period (1937–1996) was subtracted from annual values and then divided by the standard deviation of the common period for each individual core. Environmental records SST for the period of 1937–1996 was obtained from the 1°×1° gridded HadISST 1.1 dataset centered on 24.5° N and 80.5° W, which consist of blended in situ observations and satellite AVHRR (UK Meteorological Office, Hadley Centre. HadISST 1.1—Global sea-Ice coverage and SST, 1870-Present, British Atmospheric Data Center, 2006, http://badc.nerc.ac.uk/data/hadisst/ ). Annual and seasonal rainfall records were constructed from daily rainfall data collected at Tavernier, USA (24° 59′ N, 80° 31′ W) for the period of 1937–1996 (South Florida Water Management District, www.sfwmd.gov ). Ω arag from 1937 to 1996 is derived using the OAPS model [58] applied to HadISST 1°×1° SST and WOA05 monthly salinity climatologies and is driven using global atmospheric CO 2 estimates provided by Scott Doney (WHOI) with the predicted calcification response based on the first-order empirical relationship of Langdon and Atkinson [31] in which calcification rate (G, mmol CaCO 3 m −2 h −1 )=(8±1)(Ω arag −1). Climate time series data were obtained from NOAA's National Climate Data Center ( www.ncdc.noaa.gov ) and Earth System Research Laboratory ( www.cdc.noaa.gov ). The AMO index is constructed from the Kaplan SST dataset [47] and the NAO index is constructed from the difference between instrumental pressure observations between Gibraltar, Azores and southwest Iceland [48] . How to cite this article: Helmle, K. P. et al . Growth rates of Florida corals from 1937 to 1996 and their response to climate change. Nat. Commun. 2:215 doi: 10.1038/ncomms1222 (2011).